Topological crystalline metal in orthorhombic perovskite iridates Since topological insulators were theoretically predicted and experimentally observed in semiconductors with strong spin–orbit coupling, increasing attention has been drawn to topological materials that host exotic surface states. These surface excitations are stable against perturbations since they are protected by global or spatial/lattice symmetries. Following the success in achieving various topological insulators, a tempting challenge now is to search for metallic materials with novel topological properties. Here we predict that orthorhombic perovskite iridates realize a new class of metals dubbed topological crystalline metals, which support zero-energy surface states protected by certain lattice symmetry. These surface states can be probed by photoemission and tunnelling experiments. Furthermore, we show that by applying magnetic fields, the topological crystalline metal can be driven into other topological metallic phases, with different topological properties and surface states. Recent discovery of topological insulators (TIs) reveals a large class of new materials that, despite an insulating bulk, host robust metallic surface states [1] , [2] , [3] , [4] , [5] , [6] , [7] , [8] , [9] . Unlike conventional ordered phases characterized by their symmetries, these quantum phases are featured by non-trivial topology of their band structures, and remarkably they harbour conducting surface states protected by global symmetries such as time-reversal and charge conservation. More recently, it was realized that certain insulators can support surface states protected by crystal symmetry, and they are named topological crystalline insulators [10] , [11] , [12] . The rich topology of insulators in the presence of symmetries lead to a natural question: are there similar ‘topological metals’ hosting protected surface states? After the proposal of Weyl semimetal [13] , a large class of topological metals are classified [14] , which harbours surface flat bands protected by global symmetries such as charge conservation. However, an experimental confirmation of these phases is still lacking [15] . In this work, we propose that orthorhombic perovskite iridates AIrO 3 , where A is an alkaline-earth metal, with strong spin–orbit coupling (SOC) and Pbnm structure, can realize a new class of metal dubbed topological crystalline metal (TCM). Topological properties of such a TCM phase include zero-energy surface states protected by the mirror-reflection symmetry, and gapless helical modes located at the core of lattice dislocations. Photoemission and tunnelling spectroscopy are natural experimental probes for these topological surface states. We further show how this TCM phase can be driven to metallic phases with different topology by applying magnetic fields, which breaks the mirror symmetry. All these results will be supported by topological classification in the framework of K-theory, as well as numerical calculations of topological invariants and surface/dislocation spectra, as presented in the Methods section. Crystal structure and lattice symmetry in SrIrO 3 Iridates have attracted much attention due to the strong SOC in 5d-Iridium (Ir) and a variety of crystal structures ranging from layered perovskites to pyrochlore lattices [16] , [17] . Despite structural differences, a common ingredient of these iridates with Ir 4+ is J eff =1/2 states governing low-energy physics, resulted from a combination of strong SOC and crystal field splitting. Among them, orthorhombic perovskite iridates AIrO 3 (where A is an alkaline-earth metal) belongs to Pbnm space group and can be tuned into a TI [18] . A unit cell of AIrO 3 contains four Ir atoms as shown in Fig. 1a , and there are three types of symmetry plane: b-glide, n-glide and mirror plane perpendicular to axis. Each of them can be assigned to the symmetry operators as follows: Π b , Π n and Π m , as listed in the Methods section. Introducing three Pauli matrices corresponding to the in-plane sublattice ( τ ), layer ( ν ) and pseudo-spin J eff =1/2 ( σ ), the tight-binding Hamiltonian H ( k ) [18] has a relatively simple form shown in equation (6). 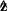Table 1 Classification of topological crystalline metals and possible surface states on a generic side surface parallel to-axis. No description available Figure 1: Crystal structure and surface states on side plane. ( a ) Crystal structure of AIrO 3 with axis along [110], axis along and axis along direction, respectively. The unit cell contains four Ir atoms: blue (B), red (R), yellow (Y) and green (G) represent different oxygen octahedra environment. The length of Bravais lattice unit vectors and axis are a / a and c , respectively. A mirror symmetry plane (coloured with light orange), mapping z to − z , locates at , where four oxygen atoms (purple solid circles) are within the same plane. ( b ) Special k -points in the 3D bulk BZ and 2D surface BZ for surface. The location of the nodal ring depict as red circles on U–R–S–X plane in 3D BZ. Slab-geometry surface spectrum ( c ) for surface at , plotted along the high-symmetry line (green dashed line) , and ( d ) for surface at k a =0 by varying k c to follow (purple dashed line), where red lines represent surface states. Full size image The band structure of tight-binding Hamiltonian H ( k ) exhibits a ring-shaped one-dimensional (1D) Fermi surface (FS) close to the Fermi level as shown in Fig. 1b , which we call the nodal ring, as the energy dispersion is linear in two perpendicular directions. This nodal ring FS was confirmed by first-principle ab initio calculations [18] , [19] , and it remains intact in the presence of Hubbard U up to 2.5 eV. Therefore, the semimetallic character of SrIrO 3 with U around 2 eV is consistent with the previous experimental results [20] , [21] . It was further shown that the size of nodal ring is determined by rotation and tilting angles of the oxygen octahedra around each Ir atom. In the case of SrIrO 3 , which has a minimal distortion of octahedra, the nodal ring is centred around the point, and extends in two-dimensional (2D) U–R–S–X plane (perpendicular to axis) in three-dimensional (3D) Brillouin zone (BZ) as shown in Fig. 1b . Zero-energy surface states and dislocation helical modes Here we show that the nodal ring FS exhibits non-trivial topology that leads to localized surface zero modes protected by the mirror symmetry, thus coined TCM. To demonstrate the existence of zero-energy surface states, the band structure calculation for the -side plane was carried out with open boundary, that is, surface perpendicular to axis. The energy dispersion at , as displayed in Fig. 1c , reveals a dispersionless zero-energy flat band marked by red colour for all k a on surface of the sample. On the other hand, the slab spectrum at k a =0 shows that the surface states are gapped except at , as shown in Fig. 1d . Similar calculations for -side plane show that [110] surface (perpendicular to axis) also supports localized surface zero modes at , while surface (perpendicular to axis) does not harbour any zero-energy states. As elaborated in the Methods section, these surface states manifest a mirror-symmetry-protected weak index labelled by a vector [22] , where and are Bravais lattice primitive vectors. A direct consequence of this weak index is the existence of zero-energy states for any side surface, except for [010] surface perpendicular to vector M . Another consequence of weak index M is the existence of pairs of counter-propagating zero modes (‘helical modes’) localized in a dislocation line, which respects mirror symmetry Π m . The number of zero-mode pairs N 0 in each dislocation line is determined by its Burgers vector B by N 0 = B · M /2 π (ref. 23 ). We have performed numerical calculations that demonstrate a pair of gapless helical modes in a dislocation line along axis with Burgers vector . Detailed results are presented in the Methods section. Classification and topological invariants To understand the topological nature of the zero-energy surface states, let us first clarify the symmetry of tight-binding model H ( k ). It turns out in the mirror-reflection-symmetric plane, H ( k ) has an emergent chiral symmetry, that is, , where . Here σ , ν and τ represent pesudo-spin space, inter-plane and in-plane sublattice, respectively. A chiral symmetry can be understood as the combination of time-reversal symmetry and certain particle-hole symmetry [24] , hence switching the sign of Hamiltonian. The presence of chiral symmetry enforces the energy spectrum of H ( k ) to be symmetrical with respect to the zero energy. It is known that chiral symmetry can protect zero-energy surface modes [25] , [26] . On the other hand, various crystal symmetries such as mirror reflection Π m bring extra non-trivial topological properties into the system we studied. Starting from the plane with mirror reflection Π m = σ z ν x and chiral symmetry , we can classify possible surface flat bands in the mathematical framework of K-theory [27] , as summarized in Table 1 (see Methods section for details). Table 1 Classification of topological crystalline metals and possible surface states on a generic side surface parallel to -axis. Full size table In particular with both mirror and chiral symmetries, the classification is characterized by a pair of integer topological invariants ( W + , W − ). Since the Hilbert space can be decomposed into two subspaces with different mirror eigenvalues Π m =±1, in each subspace we can obtain a 1D winding number [14] where k is the crystal momentum along [ lmn ] direction and is the 1D Hamiltonian parametrized by [ lmn ] surface momentum k || in Π m =±1 subspace. For both plane ([110] surface) and plane ( surface), we have ( W + , W − )=(1, −1). These quantized winding numbers correspond to a pair of zero modes for each surface momentum with , and they cannot hybridize due to opposite mirror eigenvalues. Meanwhile, for [010] surface both W ± vanish, indicating a weak index [22] . Intuitively, the system can be considered as a stacked array of planes, each plane (perpendicular to axis) with a pair of mirror-protected zero-energy edge modes at . Once the mirror symmetry Π m is broken, the classification becomes characterized by one integer topological invariant: the total winding number W ≡ W + + W − associated with 1D TI in symmetry class AIII [24] , [27] . This total winding number vanishes for all surface momenta at though. Topological metal/semimetal induced by magnetic fields Time-reversal (TR) breaking perturbations such as a magnetic field can drive the system from the TCM phase to other metallic phases with different topological properties. In the presence of Zeeman coupling μ B h · σ introduced by magnetic field h , clearly the chiral symmetry is still preserved as long as the field is in plane ( ). Magnetic field parallels to axis breaks chiral symmetry, which gaps the nodal ring, making the system trivial. Meanwhile, mirror symmetry Π m will be broken unless the magnetic field is along direction. Thus, our focus below will be magnetic field in the plane. 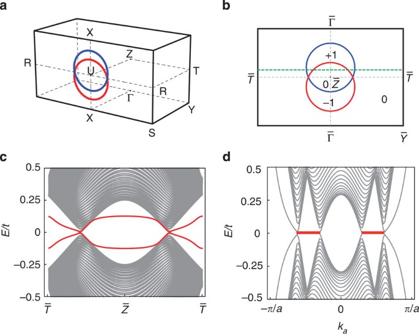Figure 2: Evolution of the nodal ring under various TR-breaking terms and corresponding surface modes. (a) When the magnetic field, a pair of nodal rings contain one ring (blue) shifted upwards alongaxis and the other one (red) shifted downwards. (b) The corresponding winding numberdistribution onplane. Slab spectrum (c) whenforsurface plotted as a function ofkaalong the high-symmetry line, and (d) whenindicated by the green dashed line in (b). The FS topology and associated surface states with a magnetic field along different directions are listed in Table 2 . Table 2 Various TR-breaking perturbations and consequences on the nodal ring and surface states (for example, on side surface). Full size table Chiral topological metal protected by chiral symmetry Due to TR and inversion symmetry, the nodal ring in TCM always has twofold Kramers degeneracy. After applying direction magnetic field , the doubly degenerate nodal ring in Fig. 1b splits into two rings in Fig. 2a shifted along axis on U–R–S–X plane. Although the mirror symmetry is broken by the magnetic field, chiral symmetry is still preserved. Therefore, the topological properties of the two nodal rings are captured by an integer winding number W in the symmetry class AIII [14] . Consider surface for instance, depending on the surface momentum k || , the winding number is plotted in Fig. 2b . It vanishes in the region where the two nodal rings (blue and red) overlap, but becomes ±1 in other regions within the two nodal rings. Figure 2: Evolution of the nodal ring under various TR-breaking terms and corresponding surface modes. ( a ) When the magnetic field , a pair of nodal rings contain one ring (blue) shifted upwards along axis and the other one (red) shifted downwards. ( b ) The corresponding winding number distribution on plane. Slab spectrum ( c ) when for surface plotted as a function of k a along the high-symmetry line , and ( d ) when indicated by the green dashed line in ( b ). Full size image The energy spectra on a slab geometry with open surfaces are displayed in Fig. 2c,d , plotted as a function of k a with and , respectively. There is no zero modes at , corresponding to trivial winding number. Meanwhile, zero-energy flat bands highlighted by red colour in Fig. 2d exist inside the nodal rings. It confirms the non-trivial topology of the bulk nodal rings with quantized winding number shown in Fig. 2b . It turns out this chiral topological metal supports localized flat band protected by chiral symmetry on any surface, as long as its normal vector is not perpendicular to axis. Meanwhile, the two nodal rings are stable against any perturbations preserving chiral symmetry, since the winding number changes when we cross each nodal ring [14] . Weyl semimetal Once we apply a magnetic field along [110] direction (or axis), both mirror (Π m ) and n-glide (Π n ) symmetries are broken. Consequently, the nodal ring is replaced by a pair of 3D Dirac nodes, appearing at momenta along the path R→U→R BZ line. However, these Dirac nodes are not symmetry protected, since a sublattice potential mν z alternating by layers would further split each Dirac point into a pair of Weyl nodes. And this mν z term has the same symmetry as a Zeeman field h [110] along axis. In the presence of both magnetic field h [110] and layer-alternating potential mν z , the system still preserves chiral symmetry , b-glide Π b and inversion symmetry. Two pairs of Weyl nodes emerge at and along R→U→ R line in Fig. 3a . 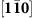Figure 3: Emergence of Weyl fermions onside surface. (a) Two pairs of Weyl node located along the high-symmetry line U→R atk1andk2, respectively. One of the Weyl fermion (blue) has +1 chirality but the other Weyl node (red) has opposite chirality. The Fermi arc connecting those two Weyl nodes is coloured by green. (b)The edge states spectra when, which is in between two Weyl nodes plotted as a function ofkc. The low-energy Hamiltonian around k 1 has linear dispersion along all k directions Figure 3: Emergence of Weyl fermions on side surface. ( a ) Two pairs of Weyl node located along the high-symmetry line U→R at k 1 and k 2 , respectively. One of the Weyl fermion (blue) has +1 chirality but the other Weyl node (red) has opposite chirality. The Fermi arc connecting those two Weyl nodes is coloured by green. ( b )The edge states spectra when , which is in between two Weyl nodes plotted as a function of k c . Full size image with δ k ≡ k – k 1 . Various coefficients can be expressed in terms of the tight-binding hopping parameters (see Methods). There exists a ‘jump’ for the Chern number C for all occupied bands from C =0 to C =1 when k a crosses k 1 , and similarly an opposite ‘jump’ from C =1 to C =0 after k a passes k 2 . The different signs of jumps in Chern number indicate that the Weyl fermions at ± k 1 and ± k 2 have opposite topological charge +1 (blue) and −1 (red), respectively, as shown in Fig. 3a . The surface states on surface at , between the two Weyl nodes with opposite chirality, are plotted along k c in Fig. 3b . There is a single dispersing zero mode coloured with red in Fig. 3b , which is localized on each surface of the sample. A series of one-way-dispersing zero modes for all surface momenta between k 1 and k 2 form a ‘chiral Fermi arc’ [13] , [28] on surface, as shown by the green lines in Fig. 3a . The existence of surface zero modes in our TCM phase originates from the chiral and mirror-reflection symmetry of AIrO 3 with Pbnm structure. Any side surface other than [010] plane should exhibit robust zero-energy surface states independent of the details. In a generic band structure of SrIrO 3 , this nodal ring does not sit exactly at the Fermi level E F , but slightly below E F (unless SOC is stronger than an atomic SOC used in the first-principle calculation), and a hole-like pocket FS occurs around Γ point in Fig. 1b [19] . In other words, the nodal ring occurs around , while the small bulk Fermi pocket is located near k c =0. Therefore, the zero-energy surface modes are well separated from the bulk FS pockets in momentum, and a momentum-resolved probe is required to detect the surface states. Angle-resolved photoemission spectroscopy (ARPES) would be the best tool to observe the momentum-resolved surface states shown in Fig. 1c,d on a side plane of AIrO 3 . Notice that, ARPES has successfully detected the topological surface states in Dirac semimetal material [29] . Due to the presence of extremely small orbital overlap amplitudes between further Ir sites, the surface states acquire a slight dispersion. However, as we emphasized above, the mirror symmetry is a crucial ingredient to support such non-trivial surface states detectable by ARPES, despite the ‘weak breaking’ of chiral symmetry. These surface states also contribute finite surface density of states (SDOSs) near zero energy. In contrast, the semimetallic bulk band contribution to SDOS vanishes around zero energy due to the presence of bulk nodal ring. Therefore, protected surface modes can be detected as a zero bias hump (finite SDOSs) in the dI/dV curve of scanning tunnelling microscopy. However, in real materials, it will be difficult to separate the contribution of the surface states to SDOS from the bulk part. On the other hand, there exists protected propagating fermion modes in dislocation lines [23] that preserves mirror symmetry. One advantage is that these topological helical modes are protected by mirror and chiral symmetries, and hence will not be destroyed by hybridization with bulk gapless excitations. In particular, counter-propagating gapless fermions show up in pairs in the dislocation core, and the number of gapless fermion pairs is given by M · B /2 π , where B is the Burgers vector of dislocation as shown in the Methods section. Unlike other gapless and dispersive bulk excitations that are extended in space, these helical fermion zero modes are localized near the dislocation core, which in hence can be detected by scanning tunnelling microscopy. Since a bulk sample of AIrO 3 such as SrIrO 3 requires high pressure to achieve the Pbnm crystal structure [30] , [31] , it is desirable to grow a film of AIrO 3 . Recently, superlattices of atomically thin slices of SrIrO 3 was made by pulsed laser deposition along [001] plane [32] . This work is a first step towards possible topological phases in iridates. Furthermore, a successful growth of film along [111] plane was also reported [33] . Thus, growing a film of AIrO3 along [110] (or ) is plausible. To confirm the proposed TCM, an ARPES study should be performed on a film of AIrO3 grown along [110] (or ), where the mirror symmetry of Pbnm structure is kept. This analysis should reveal a flat surface band near below E F . Symmetry operators and tight-binding Hamiltonian The tight-binding Hamiltonian is defined in the basis of eight component spinor , organized as [18] where B , R , R , G correspond to four sublattices. We define Pauli matrices τ and ν in terms of following sublattice rotations The full space group Pbnm is generated by (see Fig. 2 in ref. 18 ) translations T x,y,z (three Bravais primitive vectors correspond to and ) and the following three generators {Π b , Π n , Π m } where Π b (glide plane ) and Π n (glide plane ) represent two glide symmetries, while Π m is the mirror reflection and σ denotes the pseudo-spin subspace. I =Π b Π n Π m represents the inversion symmetry. The tight-binding Hamiltonian of SrIrO 3 has the following form [18] Here various coefficient functions have been defined in ref. 18 with additional term where t 1D is the inter-layer next nearest-neighbour hopping due to non-vanishing rotation and tilting in local oxygen octahedra. The crystal momentum ( k a , k b , k c ) relates to ( k x , k y , k z ) simply by The basis we use here is different with the basis in ref. 18 by a unitary rotation U k In this basis , the tight-binding Hamiltonian is related to H k by the unitary transformation U k in equation 6: Clearly in (or ) plane the non-vanishing terms in H k , as in the basis , contain only Pauli matrices ( τ x , σ z τ y ), ν y τ y and σ x,y ν x,z τ y . All these Pauli matrices anti-commute with that is, they all have chiral symmetry . However, in representation, the chiral symmetry written as K-theory classification procedure and topological invariants To understand surface states on surface for instance, let us focus on a 1D system H k in momentum space parametrized by fixed momentum and . Such a 1D system will have mirror reflection Π m =i σ z ν x in (5), as well as chiral symmetry in (12). We will classify such a gapped 1D system (since the bulk gap only closes at two points in plane) to see whether it has non-trivial topology, which may protect gapless surface states. The classification of a gapped system can be understood from classifying possible symmetry-allowed mass matrices for a Dirac Hamiltonian [27] , [34] . The mathematical framework of K-theory applies to both global symmetry and certain spatial (crystal) symmetry [35] , [36] . In 1D such a Dirac Hamiltonian can be written as with chiral symmetry mirror reflection Π m and U (1) charge conservation Q Any two symmetry generators among commute with each other. Mathematically, the classification problem corresponds to the following question: given Dirac matrix γ 1 and symmetry matrices , what is the classifying space of mass matrix γ 0 ? In particular, since each disconnected piece in classifying space corresponds to one gapped 1D phase, how many disconnected pieces does contain? Hence, the classification of gapped 1D phases with these symmetries is given by the zeroth homotopy . In the K-theory classification, if there are generators that commute with all Dirac matrices and other symmetry generators, such as U (1) charge symmetry generator Q here satisfying Q 2 =(−1) F , then we say the gapped system belong to a complex class. Otherwise, it belongs to a real class. Clearly, our case belongs to the complex class because both Q and M commute with any other matrices. For the k c = π / c plane on a generic [ xy 0] side surface parallel to axis, the full symmetry group is generated by as mentioned earlier. Note that these three symmetry generators all commute with each other while Q 2 =(−1) F . Together with Dirac matrix γ 1 , they form a complex Clifford algebra Cl 2 × Cl 2 : where the generators inside the parenthesis anti-commute with each other and commute with everything outside the parenthesis. The reason we have Cl 2 × Cl 2 is because we can block-diagonalize the k c = π tight-binding Hamiltonian with respect to their Π m (mirror reflection) eigenvalue ±1, and in each subspace the Clifford algebra is Cl 2 (two generator in the parenthesis). Now when we add the mass matrix γ 0 , the complex Clifford algebra is extended to Cl 3 × Cl 3 generated by Therefore, the classifying space of mass matrix γ 0 is determined by the extension problem of Clifford algebra Cl 2 × Cl 2 → Cl 3 × Cl 3 and we label such a classifying space as . The classification of gapped 1D phases with symmetries is hence given by There are two integer-valued topological invariants ( W + , W − ) that are 1D winding numbers [26] obtained in block-diagonalized subspace with Π m = σ z ν y =±1. Now let us start to break Π m and symmetries. When we break mirror reflection Π m (but keep ), the Clifford algebra extension problem becomes Cl 2 → Cl 3 and hence the classification is . The topological invariant is total winding number W = W + + W − . If we break but keep Π m , the extension problem is again ( Cl 1 ) 2 →( Cl 2 ) 2 and classification is trivial since If we break both and Π m symmetries, our extension problem is Cl 1 → Cl 1 which leads to a trivial classification π 0 ( C 1 )=0. Therefore, we obtain the results in Table 1. Dislocation spectrum One implication of weak index M is the existence of pairs of counter-propagating zero modes localized in a dislocation line respecting mirror symmetry Π m . The number of zero-mode pairs in each dislocation line is determined by its Burgers vector B : number of helical modes= B · M /2 π . (ref. 23 ) To check such zero modes due to dislocation line, we consider pair-edge dislocations along axis, with a pair of Burgers vectors: perpendicular to the dislocation line. The type of dislocation core is illustrated in Fig. 4a . We consider now a 3D box with periodic boundary condition in all directions (a 3D torus) so that the system does not have an open surface. Consider every unit cell (with four sublattices, two pseudo-spin species per site) as a lattice ‘site’ in Fig. 4a , then the system has hopping terms between nearest-neighbour ‘sites’ following the tight-binding Hamiltonian in equation (6). direction is still translational invariant and k z remains a good quantum number, but in plane translation symmetry is broken by the dislocation. The dislocation spectrum is obtained when there are 39 sites along axis and 15 sites along axis. The location of dislocation with Burgers vector is at (4,6), which means 4th site along axis and 6th site along axis. And the position of dislocation with Burgers vector is at (24,12). The dislocation spectrum has displayed in Fig. 4b highlighted by red colour. It shows two pairs of gapless helical modes localized on each dislocation cores. 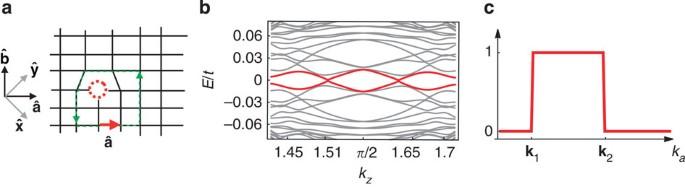Figure 4: Disloction spectrum and Chern number. (a) Top view of an edge dislocation with Burgers vector(coloured by red arrow), whose dislocation line is alongaxis. Dashed green line denotes a trajectory around the dislocation core (red circle). Clearly when we go around the dislocation once, we need an extra translation by the Burgers vector (the red arrow), equal to Bravais primitive vectorin this case) to return to the starting point. (b) The dislocation spectrum for system size 39 × 15 contains two pairs of gapless helical modes (highlighted with red colour) localized at each dislocation line. (c) Chern number as a function ofkafor all occupied bands. Opposite Chern number jump indicates that the Weyl fermion atk1andk2has different chirality. Figure 4: Disloction spectrum and Chern number. ( a ) Top view of an edge dislocation with Burgers vector (coloured by red arrow), whose dislocation line is along axis. Dashed green line denotes a trajectory around the dislocation core (red circle). Clearly when we go around the dislocation once, we need an extra translation by the Burgers vector (the red arrow), equal to Bravais primitive vector in this case) to return to the starting point. ( b ) The dislocation spectrum for system size 39 × 15 contains two pairs of gapless helical modes (highlighted with red colour) localized at each dislocation line. ( c ) Chern number as a function of k a for all occupied bands. Opposite Chern number jump indicates that the Weyl fermion at k 1 and k 2 has different chirality. Full size image Effective Hamiltonian of Weyl fermion By projecting the states around the Weyl node, the two-band Hamiltonian with linear Weyl fermion form can be obtained after adding mν z , which breaks mirror symmetry and magnetic field h [110] ( σ x + σ y ), which breaks TR symmetry to H ( k ) in equation (6). The followings are the coefficients for the effective Hamiltonian describes the Weyl fermion at k 1 of equation (2) presented in the main text: where are the coefficients in tight-binding Hamiltonian. The Chern number C for all occupied bands as a function of crystal momentum along U→R (or k a ) is shown in Fig. 4c . How to cite this article: Chen, Y. et al . Topological crystalline metal in orthorhombic perovskite iridates. Nat. Commun. 6:6593 doi: 10.1038/ncomms7593 (2015).